Atomically flat single-crystalline gold nanostructures for plasmonic nanocircuitry Deep subwavelength integration of high-definition plasmonic nanostructures is of key importance in the development of future optical nanocircuitry for high-speed communication, quantum computation and lab-on-a-chip applications. To date, the experimental realization of proposed extended plasmonic networks consisting of multiple functional elements remains challenging, mainly because of the multi-crystallinity of commonly used thermally evaporated gold layers. This can produce structural imperfections in individual circuit elements that drastically reduce the yield of functional integrated nanocircuits. In this paper we demonstrate the use of large (>100 μm 2 ) but thin (<80 nm) chemically grown single-crystalline gold flakes that, after immobilization, serve as an ideal basis for focused ion beam milling and other top-down nanofabrication techniques on any desired substrate. Using this methodology we obtain high-definition ultrasmooth gold nanostructures with superior optical properties and reproducible nano-sized features over micrometre-length scales. Our approach provides a possible solution to overcome the current fabrication bottleneck and realize high-definition plasmonic nanocircuitry. In recent years there has been considerable interest in the development of basic building blocks of optical nanocircuitry and improved photovoltaic devices that take advantage of plasmonic resonances of noble metals and the associated strongly enhanced local fields [1] , [2] , [3] , [4] . Subwavelength plasmonic waveguides [5] , [6] , optical nanoantennas [7] , [8] and various plasmonic modulators [9] , [10] and resonators for high-resolution sensing and microscopy [8] , [11] , [12] , [13] , [14] have been suggested and realized experimentally. Furthermore, the strongly enhanced local fields associated with plasmon resonances have been exploited to boost various nonlinear optical phenomena [15] , [16] . Recently, the first steps have been taken to transfer concepts of quantum optics to plasmonics [17] , [18] , [19] , [20] . In combination with coherent control techniques for near-field manipulation [21] , [22] , [23] , gain materials for field amplification [24] , [25] , [26] , [27] and the impedance matching concept for building up optical nanocircuitry [28] , [29] , functional plasmonic nanocircuitry operating at optical frequencies is becoming an important scientific and technological field. However, when it comes to advanced functional—and therefore necessarily more complex—plasmonic nanostructures, theoretical studies using numerical simulations are far ahead of what is currently within reach of state-of-the-art micro- and nanofabrication techniques [22] , [28] , [29] . This trend has roots in the very small fabrication tolerances that are necessary to yield a desired functionality. Small enough tolerances, however, are very difficult to obtain because of the multi-crystalline structure of thin gold films produced by thermal evaporation [30] . As an illustration, we consider a plasmonic transmission line consisting of two wires separated by a nanometre-sized gap extending over micrometre distances. Although such transmission lines perform well in simulations, in a real structure, fabricated by state-of-the-art nanofabrication techniques, already a single nanometre-scale defect in the gap can lead to a strong power reflection because of the local impedance change, and render the structure useless. As a general rule, fabrication tolerances become more critical as the degree of field confinement and enhancement in plasmonic nanostructures increases. For isolated nanostructures with a single critical dimension, such as the feedgap of a nanoantenna, insufficient fabrication tolerances can be compensated by producing large arrays of similar structures and selecting individuals that match specifications. This approach, however, breaks down as soon as several nanostructures, each with their own critical dimensions, need to be combined in a complex device because the yield of functional devices then decreases rapidly with the number of elements. In addition, there is clear evidence that in multi-crystalline nanostructures, scattering of plasmons is enhanced [30] , [31] , [32] , which has negative consequences for both propagation effects and the achievable maximal near-field intensity enhancement. For the progress of nanoplasmonics it is therefore crucial to have methods at hand that allow precise fabrication of complex, functional, single-crystalline plasmonic nanostructures and extended networks. When applied to the task of manufacturing complex plasmonic nanostructures, electron beam lithography (EBL), the currently most popular fabrication method, suffers from the multi-crystalline character of gold layers and ensuing imperfections introduced by the lift-off process [30] , [33] . Moreover, to enhance the sticking of very small gold nanostructures to various substrates, including indium tin oxide (ITO)-coated substrates providing DC conductivity, a standard method is to deposit a thin adhesion layer, such as 5 nm of titanium or chromium. This adhesion layer, unfortunately, damps the local plasmonic resonance drastically and thus reduces the plasmon propagation length and near-field intensity enhancement [34] , [35] , [36] , [37] . To avoid the adhesion layer, Mühlschlegel et al . [7] have chosen an approach combining EBL and focused ion beam (FIB) milling to fabricate optical nanoantennas. They first use EBL to fabricate marker structures and large gold patches (>1 μm 2 ) that, during the lift-off, stay firmly attached to the substrate even without an adhesion layer. Subsequent FIB milling then yields the desired structures. Using this approach, white-light continuum generation with very low excitation powers (down to 20 μW) has been observed for some of the antennas nominally in resonance with the excitation. As the gold film produced by vapour deposition consists of randomly oriented crystal grains, the precision of the fabricated structures is limited by the size of the grains because of the fact that different crystal domains show different resistance to FIB milling [33] . The typical diameter of crystal grains in thin layers of vapour-deposited gold is about 30–50 nm, which impedes the fabrication of structures containing features of comparable size and introduces an intrinsic surface roughness for larger structures that leads to scattering [31] and increased dephasing of surface plasmons. Alternative fabrication methods such as template stripping using a patterned silicon substrate [38] or induced-deposition mask lithography [14] retain the problem of multi-crystallinity and therefore cannot effectively remove the nanofabrication bottleneck in plasmonics. In this paper, we propose a new method for the fabrication of extended functional plasmonic nanostructures, using chemically synthesized single-crystalline gold flakes [39] , [40] , [41] that are deposited on a substrate and subsequently structured by FIB milling. Using this combination of bottom-up and top-down nanofabrication, we have obtained isolated nanoantennas and more complex plasmonic nanostructures for optical nanocircuitry with superior optical quality, well-defined dimensions and crystallographic orientation, as well as atomically flat surfaces. The use of chemically synthesized single-crystalline metal flakes is inexpensive and not limited to gold [42] . However, the chemical stability and degradation at ambient conditions may need to be taken into consideration for different metals. It can be applied to all kinds of substrates and may thus facilitate hybrid plasmonic waveguiding [6] and plasmonic lasing [27] , in which a well-controlled deep subwavelength contact between different materials is necessary. Atomically flat structures may also prove beneficial for high-precision measurements as in the area of Casimir interaction [43] , [44] , [45] and plasmonic optical trapping [46] , [47] , [48] . Properties of single-crystalline gold flakes The growth of large gold flakes is achieved following the procedure described in ref. 40 under decreased reaction temperature (see Methods ). 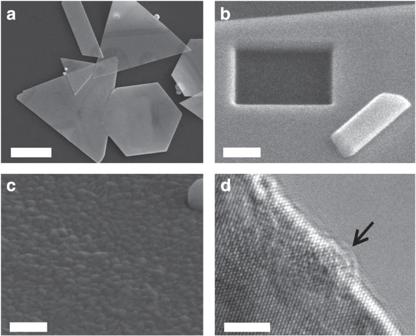Figure 1: SEM and TEM images of chemically synthesized gold flakes and vapour-deposited gold film. (a) Overview of a cluster of self-assembled single-crystalline gold flakes. The thickness of the flakes usually varies between 40 and 80 nm, but is homogeneous for each flake. Scale bar, 5 μm. (b) Zoomed-in SEM image of the surface of a single-crystalline flake with the rectangular area milled by FIB. The nearby particle is a nanoparticle from the suspension. Scale bar, 200 nm. (c) Zoomed-in SEM image of a typical surface of vapour-deposited multi-crystalline gold film (marker structure) consisting of randomly oriented grains (30–50 nm) on top of an ITO substrate. Scale bar, 200 nm. Note that (b) and (c) are recorded with a 52° tilt angle. (d) High-resolution TEM image of a single-crystalline gold flake with the edge created by FIB milling. The single-crystal domain remains after FIB milling with small particles (1–2 nm) because of redeposition of the sputtered material (black arrow). Scale bar, 2 nm. As shown in Figure 1a , single-crystalline flakes appear as triangles and truncated triangles. The high surface quality of single-crystalline flakes ( Fig. 1b ) is confirmed by both very low surface roughness (<1 nm) over a large area (1 μm 2 ) as determined by atomic force microscopy (AFM, Supplementary Fig. S1 ) and the complete absence of two-photon excited photoluminescence (TPPL) signal ( Supplementary Fig. S2 ), which is expected to be strongly enhanced in the presence of surface roughness [49] , as normally seen in a multi-crystalline metal film ( Fig. 1c ). Figure 1: SEM and TEM images of chemically synthesized gold flakes and vapour-deposited gold film. ( a ) Overview of a cluster of self-assembled single-crystalline gold flakes. The thickness of the flakes usually varies between 40 and 80 nm, but is homogeneous for each flake. Scale bar, 5 μm. ( b ) Zoomed-in SEM image of the surface of a single-crystalline flake with the rectangular area milled by FIB. The nearby particle is a nanoparticle from the suspension. Scale bar, 200 nm. ( c ) Zoomed-in SEM image of a typical surface of vapour-deposited multi-crystalline gold film (marker structure) consisting of randomly oriented grains (30–50 nm) on top of an ITO substrate. Scale bar, 200 nm. Note that ( b ) and ( c ) are recorded with a 52° tilt angle. ( d ) High-resolution TEM image of a single-crystalline gold flake with the edge created by FIB milling. The single-crystal domain remains after FIB milling with small particles (1–2 nm) because of redeposition of the sputtered material (black arrow). Scale bar, 2 nm. Full size image Thickness varies from flake to flake between 40 and 80 nm but is constant within one flake. Such constant thickness, together with the single crystallinity, allows for reproducible fabrication of complete functional plasmonic circuits or arrays of isolated structures with critical dimensions over large areas using a constant and optimized ion beam condition within a single flake. To our experience, clean gold flakes stick sufficiently well to the substrate spontaneously. Nanostructures fabricated from such flakes are robust during transportation and characterization, including optical investigations, electron beam imaging, and AFM measurements. Similar robustness was also observed in previous experiments on gold nanostructures without the adhesion layer [7] . We note that, if necessary, sticking may be improved by introducing covalent molecular linkage between suitably functionalized flakes and surfaces. Focused ion beam milling of single-crystalline gold flakes As a result, we are able to fabricate nanostructures that exhibit ultrasmooth surfaces and small gaps over extended distances, which is not possible using any other approach. Figure 1d shows a high-resolution transmission electron microscopy (TEM) image recorded at the FIB-milled edge of a single-crystalline flake on a carbon film substrate. This image indicates that the crystallinity of the gold flakes is hardly affected by the ion beam. However, surface contamination with very small (1–2 nm) particles, possibly due to redeposition of the sputtered material, is observed. Another anticipated intrinsic side effect of FIB milling is the Ga ion implantation. We have performed energy dispersive X-ray (EDX, see Methods ) analysis of gold flakes at a position close to an FIB-milled edge and the result shows no measurable Ga ion implantation, corresponding to a Ga ion concentration of less than 1% (see Supplementary Fig. S3 ). The effects of Ga ion implantation are not clear and need further investigation. Nevertheless, our method can be combined with various alternative top-down approaches, such as deposition mask lithography [14] , to avoid such possible side effects. 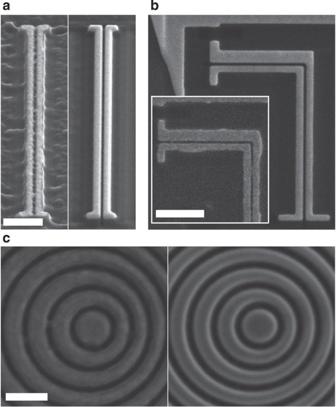Figure 2: SEM images of single- and multi-crystalline gold nanostructures. (a) Prototype optical nanocircuits22,29fabricated using FIB on a vapour-deposited multi-crystalline (left) and a single-crystalline gold flake deposited on a dip-coated ITO substrate (right). The length of nanoantennas and of the two-wire transmission line are 380 nm and 4 μm, respectively. Scale bar, 500 nm. Note that images in (a) are recorded with a 52° tilt angle. (b) Optical nanocircuits with a 90° corner fabricated with FIB on a multi-crystalline gold film, with a gap of about 28 nm between the two wires (inset) and a single-crystalline gold flake on top of a sputtered ITO substrate. Scale bar, 500 nm. (c) Asymmetric bull's eye (annular resonator) nanostructure fabricated with FIB on single- (right) and multi-crystalline (left) gold films. Scale bar, 300 nm. Note the increased roughness and structural imperfections of the multi-crystalline structures. In Figure 2 we compare the quality of nanostructures fabricated from single-crystalline gold flakes (right side of each panel) and from vapour-deposited multi-crystalline gold layers of the same thickness (left side of the panels) fabricated using the same FIB milling pattern and optimized conditions. It is evident that nanostructures with very fine features that extend over large areas can be easily fabricated in single-crystalline gold flakes. Although for multi-crystalline structures, similar structural details (for example, wire separation) can be achieved, the presence of grains leads to unpredictable structural defects, such as particles bridging the gap in Figure 2a,b . The high quality of the structures is reproducible and greatly improved compared with previously used structures [8] , [15] , [30] , [38] . In contrast to structures fabricated using vapour-deposited multi-crystalline gold films, the quality of plasmonic nanostructures obtained by our new method is independent of the surface roughness of the ITO substrate (compare Fig. 2a,b for the effect of different ITO substrates). Figure 2: SEM images of single- and multi-crystalline gold nanostructures. ( a ) Prototype optical nanocircuits [22] , [29] fabricated using FIB on a vapour-deposited multi-crystalline (left) and a single-crystalline gold flake deposited on a dip-coated ITO substrate (right). The length of nanoantennas and of the two-wire transmission line are 380 nm and 4 μm, respectively. Scale bar, 500 nm. Note that images in ( a ) are recorded with a 52° tilt angle. ( b ) Optical nanocircuits with a 90° corner fabricated with FIB on a multi-crystalline gold film, with a gap of about 28 nm between the two wires (inset) and a single-crystalline gold flake on top of a sputtered ITO substrate. Scale bar, 500 nm. ( c ) Asymmetric bull's eye (annular resonator) nanostructure fabricated with FIB on single- (right) and multi-crystalline (left) gold films. Scale bar, 300 nm. Note the increased roughness and structural imperfections of the multi-crystalline structures. Full size image Optical properties of single-crystalline gold nanostructures In the following sections, we show that our method improves not only the structural quality but also the optical properties by reducing the scattering of surface plasmons, similar to improvements observed for gold structures [31] , [50] and single-crystalline silver wires [32] . 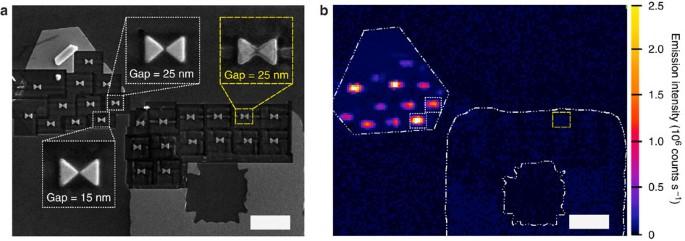Figure 3: SEM image and the corresponding TPPL map of single-crystalline and multi-crystalline gold bowtie nanoantennas. (a) SEM image of bowtie antennas fabricated by FIB using a self-assembled single-crystalline gold flake and a vapour-deposited multi-crystalline gold film with a 5 nm titanium adhesion layer on top of a sputtered ITO substrate. (b) Map of visible TPPL of the same area shown in (a), obtained by scanning the sample over the tightly focused laser spot (λ=828 nm, N.A.=1.4, average power=70 μW, pulse duration=1 ps) and recording emission intensity with a notch filter (OD >6 at 830 nm) and a band-pass filter (frequency window=450–750 nm). Scale bar, 2 μm. Figure 3a shows a scanning electron microscope (SEM) image of bowtie nanoantennas fabricated side-by-side on a single-crystalline gold flake and on a multi-crystalline gold patch prepared by EBL. Note that a 5-nm-thick titanium adhesion layer is used here for the multi-crystalline gold film representing the commonly used metal film in EBL. Figure 3: SEM image and the corresponding TPPL map of single-crystalline and multi-crystalline gold bowtie nanoantennas. ( a ) SEM image of bowtie antennas fabricated by FIB using a self-assembled single-crystalline gold flake and a vapour-deposited multi-crystalline gold film with a 5 nm titanium adhesion layer on top of a sputtered ITO substrate. ( b ) Map of visible TPPL of the same area shown in ( a ), obtained by scanning the sample over the tightly focused laser spot ( λ =828 nm, N.A.=1.4, average power=70 μW, pulse duration=1 ps) and recording emission intensity with a notch filter (OD >6 at 830 nm) and a band-pass filter (frequency window=450–750 nm). Scale bar, 2 μm. Full size image We probe the quality of plasmonic nanostructures by recording their TPPL (see Methods ). TPPL has been extensively used for the characterization of the resonant behaviour of nanoparticles [7] , [49] , [51] , [52] , [53] , [54] . The TPPL intensity is proportional to I 2 , where I is the local near-field intensity enhancement [49] , [51] , [52] . The recorded TPPL map ( Fig. 3b ) shows that, in addition to the distinct improvement of the structural quality, single-crystalline antennas show a much higher TPPL emission count rate (>100 times) upon resonant excitation, indicating much larger field enhancement. The much lower TPPL signal of the multi-crystalline antennas is attributed to the increased damping and slight resonance shift due to the adhesion layer and enhanced plasmon scattering in the multi-crystalline gold [31] . Besides, as typical materials used for adhesion layers, that is, Ti and Cr, have higher resistance to FIB milling [33] , the minimal ion dose optimized for finest spatial resolution can be insufficient to completely remove the adhesion layer in the gap. Consequently, the impedance and optical properties of nanoantennas can be strongly influenced because of the remaining material in the gap, which functions as a nanoload [28] , [55] . For the multi-crystalline bowtie antennas in Figure 3 , the excitation power needs to be increased up to 170 μW to obtain a measurable TPPL signal, as compared with <10 μW for the single-crystalline ones. This may be attributed to the fact that, according to numerical simulations, the source excitation spectrum (centred at 828 nm) does not exactly hit but only overlaps partially with the broad resonance peak of the bowtie antennas ( Supplementary Fig. S4 ). Any scattering or damping of the near field reduces the TPPL signal drastically because of the quadratic dependence of TPPL on the integrated intensity in the gold structures. Effects of the adhesion layer To disentangle the damping introduced by the adhesion layer and the damping due to increased scattering at crystal domain boundaries, we have also prepared multi-crystalline gold patches without adhesion layer using EBL. To allow for a direct comparison of single- and multi-crystalline structures, the thickness of the gold flake is reduced to 30 nm using a low-energy ion beam before writing the nanoantennas, such that the height of single- and multi-crystalline nanoantennas is nearly identical (see Methods ), as confirmed by AFM ( Supplementary Fig. S5 ). The SEM image ( Fig. 4a ) shows linear dipole antenna arrays fabricated using both a single-crystalline gold flake and the multi-crystalline gold film (marked with a white-dashed rectangle; four rows, each containing antennas with the same dimensions). On longitudinally polarized illumination (828 nm, 1 ps, 50 μW), both single- and multi-crystalline antenna arrays now exhibit easily detectable TPPL emission. Furthermore, because of the fact that the antenna length is increasing in steps of 20 nm, from left to right in the arrays (196–396 nm, respectively), a dependence of the TPPL emission rate on antenna length is observed ( Fig. 4b,c ), which reaches a maximum for those antennas the resonance of which has the best spectral overlap with the excitation source. A second maximum and the spot shape transformation related to the antibonding mode [51] are also seen. We observe that, on an average, single-crystalline antennas show much higher emission count rates even though the structural parameters of most single- and multi-crystalline antenna pairs are nearly identical. In addition to the higher count rate, the single-crystalline antenna array reproduces in a much better manner the length-dependent intensity evolution as predicted by finite-difference time-domain (FDTD) simulations. In particular, we note that some of the multi-crystalline antennas remain completely dark (yellow-dashed circle in Fig. 4 ). Checking the respective SEM images, it is observed that all dark antennas have gaps not completely cut through, possibly because of the presence of grains. It is further observed that, overall, the structural quality of single-crystalline antennas is significantly improved compared with the multi-crystalline counterparts. While many multi-crystalline antennas exhibit structural defects ( Fig. 4d , upper row), including defective gaps, single-crystalline antennas very reproducibly display homogenous structural properties, such as width, gap, shape and relative orientation of the two antenna arms. 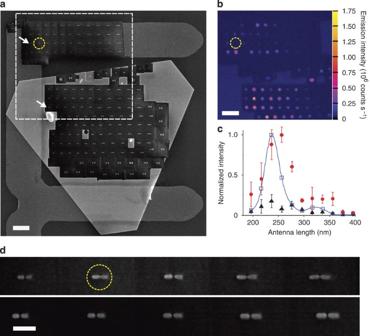Figure 4: SEM image and the corresponding TPPL map of single-crystalline and multi-crystalline linear dipole nanoantennas. (a) SEM overview image of the entire area subject to FIB milling showing a large single-crystalline gold flake and patches of a vapour-deposited multi-crystalline gold film without adhesion layer on top of a sputtered ITO substrate. The yellow circle shows a defect in the fabricated structure. Scale bar, 1 μm. (b) TPPL map of the area marked with the white-dashed rectangle in (a). Scale bar, 1 μm. (c) Averaged integrated TPPL intensity obtained from nanoantennas on single-crystalline (red dots) and multi-crystalline (black triangles) gold films in the white-dashed area in (a), plotted versus nominal antenna length, together with results obtained from the simulation (blue open squares, blue solid line is a guide for the eye). All experimental results are normalized to the maximal signal obtained from single-crystalline nanoantennas and error bars indicate the s.d. obtained from measurements on four nominally identical but distinct antenna arrays on the same flake. (d) Zoomed-in SEM images of the antenna series indicated by white arrows in (a). The yellow circle shows a defect in the fabricated structure. Scale bar, 300 nm. In particular, the examples shown in Figure 4 clearly illustrate our finding that dipole antennas fabricated from single-crystalline flakes reproducibly show the predicted length-dependent behaviour, as the gap width can be kept constant over a whole array of structures. In contrast, for a multi-crystalline gold film without adhesion layer, the gap width shows strong variations—only occasionally can structures of high quality be found. Figure 4: SEM image and the corresponding TPPL map of single-crystalline and multi-crystalline linear dipole nanoantennas. ( a ) SEM overview image of the entire area subject to FIB milling showing a large single-crystalline gold flake and patches of a vapour-deposited multi-crystalline gold film without adhesion layer on top of a sputtered ITO substrate. The yellow circle shows a defect in the fabricated structure. Scale bar, 1 μm. ( b ) TPPL map of the area marked with the white-dashed rectangle in ( a ). Scale bar, 1 μm. ( c ) Averaged integrated TPPL intensity obtained from nanoantennas on single-crystalline (red dots) and multi-crystalline (black triangles) gold films in the white-dashed area in ( a ), plotted versus nominal antenna length, together with results obtained from the simulation (blue open squares, blue solid line is a guide for the eye). All experimental results are normalized to the maximal signal obtained from single-crystalline nanoantennas and error bars indicate the s.d. obtained from measurements on four nominally identical but distinct antenna arrays on the same flake. ( d ) Zoomed-in SEM images of the antenna series indicated by white arrows in ( a ). The yellow circle shows a defect in the fabricated structure. Scale bar, 300 nm. Full size image Elastic white-light scattering As an independent proof of the fact that the single- and multi-crystalline antenna structures have almost identical dimensions and the fabricated nanoantenna arrays include nanoantennas that are on resonance with the 830 nm excitation light, we have further recorded white-light scattering spectra (see Methods ) of the nanoantennas. 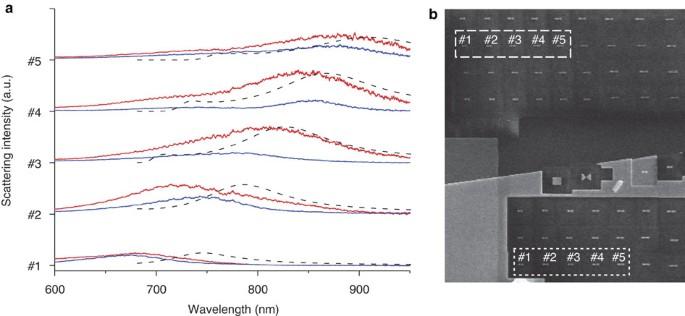Figure 5: White-light scattering spectra and simulated near-field spectra of the nanoantennas. (a) White-light scattering spectra for single-crystalline (red thick solid) and multi-crystalline nanoantennas (blue thin solid), together with simulated near-field spectra (black thin dashed) obtained using FDTD simulations. The simulated spectra are normalized to the amplitude of the single-crystalline nanoantenna spectra, and thus given in arbitrary units (a.u.). The curves are plotted with increasing offset for clarity. (b) SEM image of the corresponding single-crystalline (dotted rectangle) and multi-crystalline (dashed rectangle) nanoantennas used in (a). As shown in Figure 5 , the peak positions and widths of the selected (resonance in the visible/near-infrared) single- and multi-crystalline antennas with the same nominal dimensions are very close to each other, indicating very similar dimensions, in accordance with the AFM results. We therefore conclude that the structures that are compared have nominally the same structural dimensions and resonance frequencies. The difference in TPPL intensity can therefore be attributed to differences in the local field enhancement of the structures. Compared with the simulated spectra (black-dashed lines in Fig. 5 ), the experimental resonances seem blue-shifted. This can be attributed to the possibly larger effective gap size in the fabricated structures that results in blue-shifted spectra. We note that the agreement with simulated spectra can still be considered very good, as only small changes in the dimensions of the simulated structures would be sufficient to improve the agreement between the experiment and simulations. In Figure 5 , it is also clearly seen that single-crystalline nanoantennas show much higher scattering intensity than multi-crystalline ones, whereas the spectral line width is more or less comparable. Such higher scattering intensity is in accordance with the stronger TPPL signal and supports one of our main findings, which is that single-crystalline nanoantennas exhibit superior optical properties. Figure 5: White-light scattering spectra and simulated near-field spectra of the nanoantennas. ( a ) White-light scattering spectra for single-crystalline (red thick solid) and multi-crystalline nanoantennas (blue thin solid), together with simulated near-field spectra (black thin dashed) obtained using FDTD simulations. The simulated spectra are normalized to the amplitude of the single-crystalline nanoantenna spectra, and thus given in arbitrary units (a.u.). The curves are plotted with increasing offset for clarity. ( b ) SEM image of the corresponding single-crystalline (dotted rectangle) and multi-crystalline (dashed rectangle) nanoantennas used in ( a ). Full size image Although the comparable dimensions, that is, height, width, length and gap size, of antennas in both arrays result in a very close resonance peak position, the imperfections in the nanoantenna shape, including bumps, tilted arms and even shorted gaps, lead to worse-defined multi-crystalline antennas with lower scattering and distorted spectra. Therefore, compared with multi-crystalline antennas, single-crystalline antennas may have lower non-radiative decay rate because of the single crystallinity [56] but higher radiative decay rate because of a better defined shape. However, because of the additional geometrical factors, the observed line width and scattering amplitude cannot be intuitively understood as different contributions to the total decay rate cannot be easily disentangled. A quantitative comparison of the observed line widths is interesting but not straightforward and needs further systematic study. Compared with single-crystalline gold layers prepared by the Czochralski process and subsequent polishing [31] , [50] , or the epitaxial growths of gold layers on lattice-matched substrates such as mica or MgO, the method proposed here using chemically synthesized gold flakes is easier, cheaper and requires no specialized instrumentation while the freedom of choosing a substrate at will is retained. The obtained metal layers have well-defined crystal orientation and very large aspect ratio. The large flake area, single crystallinity and constant thickness within one flake facilitate reproducible top-down fabrication and render precise positioning of the flake on a substrate unnecessary. However, promising nanoparticle alignment techniques [57] , [58] and nanomanipulation [59] have been reported and may be applied to gold flakes as well. In addition, as the crystal orientation can be directly identified from the shape of the flakes, nanostructures can be easily fabricated with distinct crystal orientations determined by the orientation of the FIB milling pattern with respect to the single-crystalline gold flake. This would allow a direct measurement of the optical properties of nanostructures as a function of the crystal orientation. In conclusion, we demonstrate a new method for the FIB fabrication of single-crystalline plasmonic nanostructures using large and thin chemically grown single-crystalline gold flakes deposited onto a glass/ITO surface. This combination of bottom-up and top-down nanofabrication yields greatly improved fabrication tolerances, as well as improved structural homogeneity compared with conventional multi-crystalline structures. We are therefore able to fabricate plasmonic gold nanostructures with reproducible and well-defined nanometre-scale features extending over micrometre-length scales. We demonstrate the improved optical quality of our structures by means of the enhanced TPPL emission of single-crystalline linear dipole and bowtie optical antennas, which serve as a benchmark for their strong near-field intensity enhancement. Our method provides possible solutions for the fabrication and realization of high-definition complex plasmonic nanodevices and extended optical nanocircuits, as well for precise measurement of nanoscale strong interaction forces. Flake fabrication and sample preparation The growth of large gold flakes is achieved following the procedure described in ref. 40 . The reaction temperature has been reduced to 60 °C ( Supplementary Fig. S6 ) to obtain thin flakes (thickness <80 nm) with a large surface area (>100 μm 2 ). The produced gold flake suspension is rinsed and stored as an aqueous suspension. We note that further processing of the rinsed suspension, such as centrifuging or filtering, may help to remove unwanted small particles but also decreases the yield of the flakes. Ultrasonication for 5 min is used to homogeneously disperse the gold flakes before directly drop-casting the suspension onto ITO-coated coverglasses, on which multi-crystalline gold marker structures with 30 nm thickness are prefabricated by EBL. After the solvent dries out, flakes with a sufficiently large area and homogeneous contact with the substrate are preselected using a wide-field optical microscope with a low-magnification air objective (×20). The preselected flakes are then double checked with SEM, wherein the homogeneity of image brightness is used as a positive indicator. The marker structures are designed to be easily observable in both conventional optical microscopy and SEM, thus facilitating the precise localization and identification of the same gold flakes using both methods ( Supplementary Fig. S7 ). In addition, vapour-deposited markers provide multi-crystalline gold films for control experiments. Focused ion beam milling FIB milling (Helios Nanolab, FEI Company) is applied to single-crystalline flakes that pass all those criteria and are found near multi-crystalline marker structures serving as a reference. Best structuring results are obtained for 30 kV acceleration voltage and 1.5 pA Ga ion current. Although the same FIB patterns and settings are used to fabricate the structures, the ion-beam dose is optimized for the multi- and single-crystalline areas, respectively, so that the finest features, for example, the gap size of nanoantennas or the width of a linear cut, are comparable. The distance between adjacent structures is larger than 700 nm to minimize crosstalk and to ensure that only one structure is illuminated by the focal spot (full-width at half-maximum=360 nm). Using these settings, writing arrays of linear nanoantennas/bowties covering an area of 10×10 μm usually takes less than 1 h. Before starting the antenna fabrication, the flake was thinned down to match the thickness of the multi-crystalline marker structure (30 nm). For fabrications of both single- and multi-crystalline antennas, FIB milling removes 20–25 nm of ITO layer, which results in a topography contrast of about 55–60 nm from the milled ITO surface to the antenna upper surface ( Supplementary Fig. S5 ). Such geometrical details are taken into consideration in the numerical simulations. Energy dispersive X-ray analysis EDX analysis was performed at the patterned edge of the nanostructure with an FEI Titan 80–300 TEM equipped with a retractable X-ray detector (EDAX). The sample was prepared by deposition of single-crystalline gold flakes on a thin carbon film. A suitable flake was identified and patterned by a focused Ga ion beam in a dual-beam system (Helios Nanolab, FEI Company). The sample was then transferred to the TEM, which was operated at a 300 kV acceleration voltage and a beam current of 1 nA. Under these conditions, the beam diameter is around 1 nm. The sample was tilted by 10 degrees towards the detector to increase the count rate. After imaging the sample in scanning mode using a high-angle annular dark field detector, the beam was positioned at the edge of a cut in the gold flake, and the X-ray spectrum ( Supplementary Fig. S3a ) was recorded with a width of 5 eV per channel and 64 s integration time. The energy resolution of the detector was 129 eV at 5.9 keV X-ray energy. The Fe, Co and Cu lines visible in the spectrum are due to electrons that are scattered by the sample and that hit the TEM column, the pole piece of the objective lens or the copper support grid of the carbon film. To quantify the upper limit of Ga at the edge of the gold flake, we recorded the X-ray spectrum of a reference sample (gold-coated GaAsP nanowire) that was also deposited on a carbon film ( Supplementary Fig. S3b ). The spectrum of the reference sample was analysed using the TEM Imaging and Analysis software package from FEI. The compositional analysis of the reference sample (excluding the Fe, Co and Cu peaks) was then related to the count rates in the energy range where the Ga peak showed up (9–9.4 keV). Two-photon photoluminescence imaging To obtain a TPPL intensity map, the ultrashort pulses from a mode-locked Ti:sapphire laser (centre wavelength=828 nm, 80 fs, 80 MHz, Time-Bandwidth Products, Tiger) are coupled into 1.5 m of optical fibre to be stretched to approximately 1 ps. The linear polarized fibre output is then collimated, passed through a dichroic mirror (DCXR770, Chroma Technology) and focused through the coverglass onto the nanostructures using an oil immersion microscope objective (Plan-Apochromat ×100, Oil, N.A.=1.4, Nikon). The direction of the linear polarization of the beam is adjusted using a λ/2 waveplate. The photoluminescence signal is collected by the same objective and reflected by the dichroic mirror. Laser scattering and possible second harmonic signals are rejected by a holographic notch filter (OD >6.0 at 830 nm, Kaiser Optical System) and a band-pass filter (transmission window: 450–750 nm, D600/300, Chroma Technology) in front of the photon detector (SPCM-AQR 14, Perkin-Elmer). The polarization ( Supplementary Fig. S8 ) and power dependence ( Supplementary Fig. S9 ) behaviour, together with the emission spectrum of the photoluminescence ( Supplementary Fig. S2 ), confirms that the signal recorded for Figure 4c is mainly TPPL due to excitation of the longitudinal resonance of the nanoantennas. Atomic force microscopy AFM measurements are taken under ambient conditions with tapping mode operating at a resonance frequency of 240–280 kHz and a scanning rate of 0.2 Hz (DMLS scanning head, Nanoscope IIIa, Digital Instruments). White-light scattering spectroscopy To obtain white-light scattering spectra, an off-axis and s-polarized needle-like beam (collimated beam with 1–2 mm diameter) obtained from a halogen lamp (Axiovert, Zeiss) with polarization along the long axis of the antenna is focused by a microscope objective (Plan-Apochromat, 63, N.A.=1.4, Zeiss) to the sample plane. As the off-axis beam is parallel to but displaced from the objective optical axis such that it hits the surface at an angle larger than the critical angle, it undergoes total internal reflection at the sample plane. Nanoantennas that are illuminated scatter light into a broad angular range collected by the same objective while the reflected excitation beam is blocked by a small beam stop in the detection path. An achromatic λ/2 waveplate and a polarizer (Glan-Thompson calcite polarizer) are used to select the polarization of the scattered light before the entrance slit (200 μm) of the spectrometer (ACTON SpectraPro 2300i, 150 grooves per mm grating blazing at 500 nm). The typical acquisition time of the charge-coupled device is 20 s. All spectra are normalized taking into account the source spectrum and the overall transmission efficiency of the optical system. Numerical simulations Numerical simulations adopting the nominal antenna dimensions used in FIB milling are performed with a commercial FDTD (FDTD Solutions v6.5.8, Lumerical Solutions). As the antenna response is sensitive to the local index of refraction, the geometry changes of the substrate due to FIB milling are taken into account. The dielectric constant of gold is modelled according to experimental data [60] and the minimal mesh size is set to 1 nm 3 . Structures are made of gold and placed on top of an ITO layer (thickness=100 nm). All boundaries of the simulation box are set to be at least 700 nm away from the structure to avoid spurious absorption of the near fields. Corners of the antenna arms are rounded in the simulations using cylinders with 10 nm diameter. To mimic the experimental conditions, the source is set to have the same spectral width as the laser used in the experiment (821–835 nm) and is focused onto the gold/ITO interface using a thin lens (N.A.=1.4) approximated by a superposition of 200 plane waves. The impulse spectrum is recorded at the centre of the feedgap and normalized to the source spectrum, whereas the total electric field intensity (|Ex| 2 +|Ey| 2 +|Ez| 2 ) distribution inside both antenna arms is recorded using 3D field profile monitors. A quantity proportional to the TPPL signal is obtained by integrating the square of the field intensity (∫∫∫{|Ex| 2 +|Ey| 2 +|Ez| 2 } 2 dxdydz) over the volume of the antenna arms [51] . How to cite this article: Huang, J.-S. et al . Atomically flat single-crystalline gold nanostructures for plasmonic nanocircuitry. Nat. Commun. 1:150 doi: 10.1038/ncomms1143 (2010).